Role of mid-gap states in charge transport and photoconductivity in semiconductor nanocrystal films Colloidal semiconductor nanocrystals have attracted significant interest for applications in solution-processable devices such as light-emitting diodes and solar cells. However, a poor understanding of charge transport in nanocrystal assemblies, specifically the relation between electrical conductance in dark and under light illumination, hinders their technological applicability. Here we simultaneously address the issues of 'dark' transport and photoconductivity in films of PbS nanocrystals, by incorporating them into optical field-effect transistors in which the channel conductance is controlled by both gate voltage and incident radiation. Spectrally resolved photoresponses of these devices reveal a weakly conductive mid-gap band that is responsible for charge transport in dark. The mechanism for conductance, however, changes under illumination when it becomes dominated by band-edge quantized states. In this case, the mid-gap band still has an important role as its occupancy (tuned by the gate voltage) controls the dynamics of band-edge charges. Semiconductor nanocrystals (NCs) fabricated by chemical [1] and physical [2] methods have been considered promising materials for applications in solution-processable devices including light-emitting diodes [3] , [4] , [5] , field-effect transistors (FETs) [6] , [7] , [8] , [9] , [10] , [11] ,photodetectors [12] , and solar cells [13] , [14] , [15] , [16] , [17] , [18] . In addition to processability from solutions, NCs are attractive because of a variety of novel physical properties that can be controlled by NC dimensions, shapes, and internal structure [19] . Several recent examples have also demonstrated a large promise of NCs for the realization of generation-III photovoltaics by employing concepts such as multiexciton generation through carrier multiplication [20] , [21] , [22] , [23] , [24] , and hot-electron extraction [25] , [26] . A significant problem in realizing practical NC-based devices is poor understanding of charge transport in NC films. Traditional assumption is that electrical conductance in NC-based structures is mediated by a network of overlapping band-edge quantized states [20] , [27] . However, recent demonstrations of a dramatic effect of surface treatments on 'dark' conductivity ( σ 0 ) of NC films [9] , combined with observations of relatively weak sensitivity of σ 0 to NC size polydispersity [10] , suggest the involvement of intra-gap states (probably of surface origin) in charge transport. Furthermore, previous FET studies have indicated that changes in the occupancy of surface traps might be responsible for observed changes in apparent levels of doping of NC films [11] . Whereas it is typically difficult to assess the nature of states involved in 'dark' charge transport, a photoresponse should involve quantized states, as these states get populated as a result of light absorption. The relative contribution of quantized states to photoconductivity compared with the states that dominate 'dark' charge transport is unclear. For example, the studies of NC photovoltaics indicate that although the open circuit voltage ( V oc ) does scale with NC band-gap energy ( E g ), it is always appreciably lower than the ideal V oc calculated for a given E g (refs 14 , 15 , 17 , 27 ) (see Supplementary Information for discussion on semiconductor bandgap and open-circuit voltage). This might be considered as an indication of a mixed character of photoconductivity, which could involve both quantized and surface-related states. One hurdle in elucidating the nature of electronic states responsible for conduction in dark and under illumination arises from the fact that the data on 'dark' transport and photoconductivity are normally obtained using different types of devices that are, respectively, three-terminal FETs, and two-terminal photodetectors or photovoltaic cells. Here we investigate the roles of quantized band-edge and intra-gap states in NC-film conductance by using three-terminal PbS–NC-based optical FETs (OFETs). We simultaneously address the problems of 'dark' transport and photoconductance, and elucidate the roles of equilibrium charges injected by applying gate voltage versus non-equilibrium carriers generated by photoexcitation. Spectrally resolved studies of a gate-voltage-dependent photocurrent reveal the existence of mid-gap states in NC films that form a weakly conducting band (mid-gap band or MGB), which serves as a charge conduit in dark. We also observe that the nature of charge transport changes under illumination when it becomes dominated by carrier migration through the network of band-edge quantized states, which is characterized by much higher mobility than the MGB. The MGB still has an important role in the photoresponse as its occupancy controls the photoconduction by controlling recombination dynamics of band-edge charges. The analysis of the gate-voltage dependence of photoresponses indicates that lifetimes of band-edge electrons are much shorter than those of holes indicating a much greater probability of electron capture at MGB states compared with holes. This suggest that photoconductivity in our films is dominated by photogenerated holes. 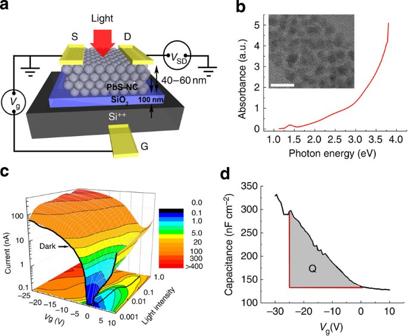Figure 1: Dark conductance and photoconductance in PbS NC OFETs. (a) A schematic of PbS–NC OFETs. S, D and G denote source, drain and gate electrodes, respectively. Illumination of PbS–NC films results in photoinduced current between the source and the drain electrodes, which is monitored as a function of light intensity and energy of incident photon, while simultaneously varying the gate voltage. (b) Absorption spectrum of PbS NCs in solution. The band-edge 1S peak is at 1.3 eV. The inset shows a representative transmission electron micrograph of the NCs (scale bar represents 10 nm). The mean NC diameter is 3.3±0.6 nm. (c) TheIsdversusVgcharacteristic in dark (black curve) and under 2.25 eV illumination as a function of light intensity (relative units; 1 corresponds to 30 μW cm−2) in a three-dimensional representation. Light illumination results in increased carrier concentration and a resultant orders-of-magnitude increase in photocurrent at the flat-band gate voltage (Vg=Vgmin; corresponds to the photocurrent minimum) due to the photoconductive effect. Under illumination, an extra positive voltage, which compensates for the photovoltage due to charge accumulation under the source/drain electrode, is required to achieve the flat-band condition (traced by the black line in the contour plot at the bottom). (d) Capacitance measurements for the NC film in dark indicate accumulation of holes in the channel under negative gate bias. The magnitude of the accumulated charge can be inferred from the integral. 'Dark' charge transport in NC films The layout of the OFET devices used in the present study is shown schematically in Figure 1a (fabrication details in Methods). Its channel is fabricated from PbS NCs with a mean diameter of 3.3 nm ( Fig. 1b inset). The corresponding band-gap energy E g =1.3 eV. First, we characterize these structures in dark (black curve in Fig. 1c ) by monitoring the source–drain current ( I sd ) as a function of gate bias ( V g ). When V g =0 (flat-band condition in our devices in dark), the OFET channel is only weakly conductive. However, I sd quickly increases under negative gate bias, which corresponds to injection of holes into the NC film. At V g =−25 V, I sd becomes ca. three orders of magnitude higher than at V g =0. From gate-source capacitance measurements ( Fig. 1d ), we estimate that that the average number of holes injected per NC ( n 0 ) at V g =−25 V is n 0 ≈0.1 (Methods). Figure 1: Dark conductance and photoconductance in PbS NC OFETs. ( a ) A schematic of PbS–NC OFETs. S, D and G denote source, drain and gate electrodes, respectively. Illumination of PbS–NC films results in photoinduced current between the source and the drain electrodes, which is monitored as a function of light intensity and energy of incident photon, while simultaneously varying the gate voltage. ( b ) Absorption spectrum of PbS NCs in solution. The band-edge 1S peak is at 1.3 eV. The inset shows a representative transmission electron micrograph of the NCs (scale bar represents 10 nm). The mean NC diameter is 3.3±0.6 nm. ( c ) The I sd versus V g characteristic in dark (black curve) and under 2.25 eV illumination as a function of light intensity (relative units; 1 corresponds to 30 μW cm −2 ) in a three-dimensional representation. Light illumination results in increased carrier concentration and a resultant orders-of-magnitude increase in photocurrent at the flat-band gate voltage ( V g = V gmin ; corresponds to the photocurrent minimum) due to the photoconductive effect. Under illumination, an extra positive voltage, which compensates for the photovoltage due to charge accumulation under the source/drain electrode, is required to achieve the flat-band condition (traced by the black line in the contour plot at the bottom). ( d ) Capacitance measurements for the NC film in dark indicate accumulation of holes in the channel under negative gate bias. The magnitude of the accumulated charge can be inferred from the integral . Full size image Although I sd also appears to increase considerably on applying the positive gate-source voltage, this growth is an artefact of our measurements, in which we switch the sign of V g without changing the sign of the source–drain voltage. As a result, the gate-drain voltage for V g >0 is considerably higher (varies from +25 V to +35 V) than in the case of V g <0 (varies from +25 V to 0), which might lead to a significant gate leakage current for positive gate voltages. This effect is likely responsible for the increase of I sd when V g >0, but not electron injection. The reason for performing the measurements without changing the sign of V sd is that the exposure of OFETs to light leads to changes in the flat-band voltage. Because of this effect, an extra positive gate voltage is required to achieve the flat-band condition on illumination. From the data in Figure 1c , however, it is still possible to evaluate the relative efficiencies of electron and hole injection into the NC channel. Specifically, because of symmetry between the gate and source electrodes (both are fabricated from gold), the conditions for hole injection at V g =−25 V are equivalent to conditions for electron injection at V g =0 V. A significantly smaller dark current measured in the latter case indicates that electron injection in our devices is much less efficient (likely negligible) than hole injection. The capacitance measurements ( Fig. 1d ) also do not show any detectable electron injection in our structures in the range of V g >0. Spectrally resolved photoresponses of OFETs Illumination of these devices with monochromatic light leads to a dramatic increase in I sd even at low light intensities, as illustrated by the three-dimensional plot in Figure 1c , for incident fluxes from 120 nW cm −2 to 30 μW cm −2 (2.25 eV illumination). The respective densities of photogenerated charges can be estimated from the product of the generation rate ( G ) and the carrier lifetime ( τ ), which yields ca 10 −4 to 10 −6 per NC for the maximum photon flux (Methods). This density is orders of magnitude lower than the number of charges injected into the film by applying a gate voltage (for example, n 0 ≈0.1 for V g =−25 V). Therefore, the fact that exposure to light leads to a dramatic increase in conductivity implies that photogenerated charges are characterized by much higher mobilities than equilibrium background charges. This strongly suggests that the natures of electronic states involved in charge transport in dark and under illumination are different. Light illumination also results in the apparent, intensity-dependent shift of the flat-band voltage traced by the black line in the contour plot at the bottom of Figure 1c . This is a reflection of the photovoltaic effect due to accumulation of photogenerated carriers under the source/drain electrode, which changes the total gate bias and hence the source–drain current (light acts as the 'fourth terminal' in our OFETs). As a result, under illumination an extra positive voltage is required to achieve the flat-band condition and the magnitude of this excess bias can serve as a measure of the photovoltaic effect. To gain further insights into the origin of charge-transporting states, we investigate the V g -dependence of photocurrent spectra that are derived from the I sd -versus- V g characteristics measured for different excitation wavelengths ( Figs 2a and b ). Under zero gate bias, the photocurrent spectrum (blue curve in Fig. 2c ) reproduces a general behaviour of a linear absorption spectrum ( Fig. 1b ) and specifically exhibits a similar spectral onset at ~1.3 eV. Application of negative V g leads to an overall increase in the photocurrent across the entire spectrum. The most striking effect of gate voltage, however, is the development of new spectral features at ~0.9 eV ( M 1S ) and ~1.5 eV ( M X ). The fact that the M 1S -band is located in the region of nominal transparency of the NC films (~0.4 eV below the 1S band-edge peak) points towards the involvement of MGB states. Further, as MGB states only manifest under negative bias, this suggests that at V g ≥0 they are fully occupied with electrons. However, some of these states become depopulated under negative V g , when the Fermi level shifts below the MGB edge. The introduction of holes into the mid-gap states unblocks optical transitions from the valence-band to the MGB levels (solid arrows in Fig. 3a ). The M 1S feature is likely associated with the transition involving the 1S h valence-band state, whereas the M X peak is probably due to some lower-lying level (labelled X h in Fig. 3a ). Because of mirror symmetry between the valence and the conduction bands in PbS [28] , [29] , the band-to-band X h – X e optical transition is expected to be located ~1.2 eV to the blue from the 1S peak, which is twice the M 1S – M X separation (~0.6 eV). Indeed, the second derivative of the absorption spectrum of the solution sample (inset of Fig. 2b ) shows a pronounced feature at ~2.5 eV, which is ~1.2 eV higher than the band-edge peak. More examples that illustrate the development of extra MGB-related spectral features in the photocurrent under negative V g are given in Supplementary Figure S1 . 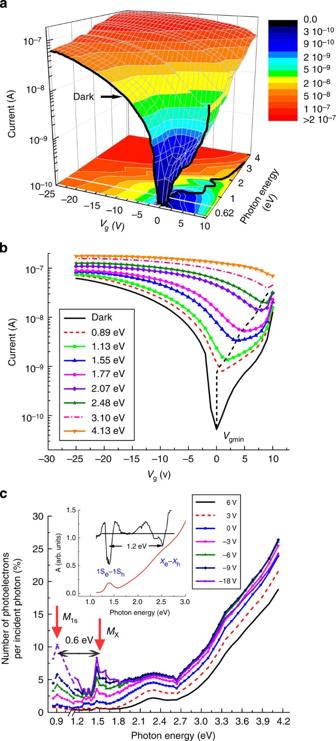Figure 2: Spectrally resolved responses of OFET indicate presence of mid-gap states forming weakly conductive band. (a)Isd-versus-Vgcharacteristics obtained in dark (black line) and under illumination as a function of photon energy starting from 0.62 eV (white line in the contour plot at the bottom). Coloured filling below the white line is interpolation between the measurements in dark and under 0.62 eV illumination. Black line in the contour plot at the bottom traces changes in the flat-band potential. (b) 'Cross-sections' obtained from the three-dimensional plots in panel 'a' show the variation of the source–drain current as a function of gate voltage under illumination at different photon energies (shown in the legend). (c) Photocurrent as a function of incident photon energy shown in terms of the number of photoelectrons per 100 incident photons (derived from data in panel 'a'). The spacing between the two prominent features (M1SandMX), that develop under negative bias, is half of the spacing between the 1S and X features in the second-derivative of the absorption (A) spectrum (inset). This suggests that the M1Sand the MXpeaks are likely due to transitions between the occupied 1S and X valence band states and the unoccupied MGB states, respectively. Figure 2: Spectrally resolved responses of OFET indicate presence of mid-gap states forming weakly conductive band. ( a ) I sd -versus- V g characteristics obtained in dark (black line) and under illumination as a function of photon energy starting from 0.62 eV (white line in the contour plot at the bottom). Coloured filling below the white line is interpolation between the measurements in dark and under 0.62 eV illumination. Black line in the contour plot at the bottom traces changes in the flat-band potential. ( b ) 'Cross-sections' obtained from the three-dimensional plots in panel 'a' show the variation of the source–drain current as a function of gate voltage under illumination at different photon energies (shown in the legend). ( c ) Photocurrent as a function of incident photon energy shown in terms of the number of photoelectrons per 100 incident photons (derived from data in panel 'a'). The spacing between the two prominent features ( M 1S and M X ), that develop under negative bias, is half of the spacing between the 1S and X features in the second-derivative of the absorption ( A ) spectrum (inset). This suggests that the M 1S and the M X peaks are likely due to transitions between the occupied 1S and X valence band states and the unoccupied MGB states, respectively. 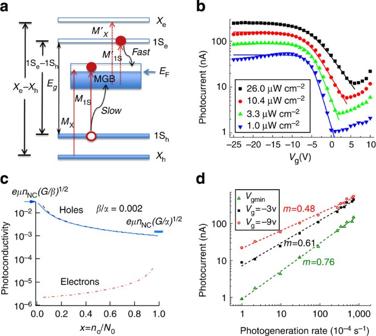Figure 3: Effect of MGB occupancy on photoconduction. (a) The energy level diagram illustrating optical transitions between the NC-quantized and MGB states (red arrows) as well as relaxation pathways (wavy black arrows) for photogenerated band-edge carriers. The blue arrow marks the position of the Fermi level (EF). (b) Photocurrent measured at different gate voltages (symbols) for light intensities from 1.04 to 26.1 μW cm−2(indicated in the figure legend) using 2.25 eV illumination. Lines are calculations using equations (4) and (5). In the modelling, the excitation intensity was characterized by the dimensionless quantityg=G/(βN02). On the basis of the photocurrent measured at large negativeVgfor 26.1 μW cm−2(solid black squares),gwas determined to be 1.3×10−3. For other traces,gwas obtained by scaling this value according to light intensity used in the measurements. γ andV0were adjustable parameters determined from the fits. The obtained values systematically varied from 0.016 to 0.007 (±0.001) forγand from 2 to 6 V (±0.15 V) forV0with increasing light intensity. (c) Calculated photoconductivity due to electrons (dashed-and-doted red line) and holes (dashed black line) using equation (3) and assuming thatxis within the interval from 0.05 to 0.95. Solid blue line is the hole photoconductivity obtained using equation (4). The arrows mark the hole-only (left) and electron-only (right) photoconductivities in the limits ofx=0 andx=1, respectively. (d) The dependence ofIsdon photogeneration rate for different gate voltages (3.1 eV photon energy). As expected for a transition from bimolecular to linear recombination, the log–log slope of this dependence is ~0.5 for the large negative gate bias (MGB is completely empty) and approaches unity as the gate bias gets more positive (MGB becomes populated). Full size image Figure 3: Effect of MGB occupancy on photoconduction. ( a ) The energy level diagram illustrating optical transitions between the NC-quantized and MGB states (red arrows) as well as relaxation pathways (wavy black arrows) for photogenerated band-edge carriers. The blue arrow marks the position of the Fermi level ( E F ). ( b ) Photocurrent measured at different gate voltages (symbols) for light intensities from 1.04 to 26.1 μW cm −2 (indicated in the figure legend) using 2.25 eV illumination. Lines are calculations using equations (4) and (5). In the modelling, the excitation intensity was characterized by the dimensionless quantity g = G /( βN 0 2 ). On the basis of the photocurrent measured at large negative V g for 26.1 μW cm −2 (solid black squares), g was determined to be 1.3×10 −3 . For other traces, g was obtained by scaling this value according to light intensity used in the measurements. γ and V 0 were adjustable parameters determined from the fits. The obtained values systematically varied from 0.016 to 0.007 (±0.001) for γ and from 2 to 6 V (±0.15 V) for V 0 with increasing light intensity. ( c ) Calculated photoconductivity due to electrons (dashed-and-doted red line) and holes (dashed black line) using equation (3) and assuming that x is within the interval from 0.05 to 0.95. Solid blue line is the hole photoconductivity obtained using equation (4). The arrows mark the hole-only (left) and electron-only (right) photoconductivities in the limits of x =0 and x =1, respectively. ( d ) The dependence of I sd on photogeneration rate for different gate voltages (3.1 eV photon energy). As expected for a transition from bimolecular to linear recombination, the log–log slope of this dependence is ~0.5 for the large negative gate bias (MGB is completely empty) and approaches unity as the gate bias gets more positive (MGB becomes populated). Full size image In the case of a fully or partially occupied MGB, one might also expect to see the transitions that promote the MGB electrons into the unoccupied conduction-band states (red-dashed arrows in Fig. 3a ). Although such transitions may indeed exist, their relative contribution to the photocurrent is much smaller than that due to the M 1S and M X features because, as discussed in detail below, the electron lifetimes in these structures are much shorter than the hole lifetimes due to a higher probability of electron capture at the MGB states. The observed spectral features due to the MGB are wider (~0.5 eV) than the 1S absorption peak (~0.2 eV). This difference is likely due to the fact that in addition to NC size-polydispersity, random NC-to-NC differences in the positions of the mid-gap levels and a systematic variation in the local Fermi level in the NC channel along the source–drain direction also contribute to the linewidths of the M 1S and M X bands. An interesting feature of the photocurrent spectra recorded under negative gate bias is the large amplitude of the MGB-related bands, which is comparable to that of the features due to intrinsic band-edge transitions. This is somewhat surprising given that the oscillator strength of the intrinsic NC transitions is expected to be stronger than for transitions involving surface-related MGB states that have a reduced spatial overlap with the wave functions of the quantized levels. However, in addition to the oscillator strength, the contribution of a given optical transition to photocurrent depends on the relative fraction of photogenerated electron-hole pairs that experience spatial separation (characteristic time τ sep ) before recombination compared with the fraction of charges that recombines geminately at or near the photogeneration site (characteristic time τ eh ). This contribution can be characterized in quantitative terms by the ratio χ = τ eh / τ sep , assuming that it is smaller than unity. It is natural to expect that the electron-hole pairs generated in intrinsic NC states have a shorter geminate recombination time and a longer charge-separation time compared with the electron-hole pairs produced through the MGB-related transitions, because the latter are characterized by a certain degree of spatial separation immediately following photogeneration. As a result, the transitions involving the MGB, although, perhaps, not as pronounced in optical absorption spectra, can still provide a significant contribution to photocurrent due to the enhanced value of χ compared with transitions involving the quantized states. The films fabricated from as-prepared NCs do not show any gating effect. This implies that the mid-gap states are likely introduced by ligand-exchange procedures, which further suggests that these states are possibly of surface origin. The MGB has a role of charge conduit under dark and its conductivity is controlled by gate bias. The MGB can be either insulating (if it is completely filled or empty) or conductive (if filled partially). In the latter case, transport through MGB can be explained in terms of either electron or hole conductivity depending on whether the Fermi level is near the bottom or the top of the MGB, respectively. This might explain the possibility of facile switching the conductivity of NC films between n - and p -type through relatively simple chemical or heat treatments [7] , [8] , [9] , [10] , [11] , [30] . In our films, under the flat-band condition, the Fermi level is located near the top of the MGB, and therefore, at V g =0 this band is essentially nonconductive. Application of negative gate bias shifts Fermi level deeper inside the MGB, which generates an increasing amount of MGB holes and results in a sharp increase of dark conductivity observed in Figure 1c . While in dark, MGB serves as a charge conduit, its role is different in the case of photoconduction. Specifically, our observation of a dramatic enhancement of I sd under illumination suggests that transport of photogenerated charges is mediated by intrinsic quantum-confined NC states that form a more conductive network, because of a greater extent of overlapping electronic wave functions compared with surface-related MGB states. The fact that, even in this case, channel conductance is sensitive to changes in gate voltage can be explained by the effect of MGB occupancy on recombination dynamics of band-edge carriers, as elaborated in the Discussion section. According to our earlier estimations, the densities of photogenerated charges ( n and p for electrons and holes, respectively) are much smaller than 1 per NC, while the density of mid-gap states ( N 0 ) is at least on the order of 1 because they form a percolated conductive network. Because p, n ≪ N 0 , the relaxation of photogenerated carriers is dominated not by band-to-band recombination but trapping at the mid-gap levels. From charge neutrality, the density of non-equilibrium electrons in the MGB under photoexcitation is n m = p − n . Alternatively, the effect of photoexcitation on occupancy of MGB states can be characterized in terms of photogenerated holes with density p m = n − p . Under steady state, the trapping rates are equal to the photogeneration rate: where α and β are electron- and hole-capture coefficients, respectively. When MGB is completely empty ( n 0 =0), equations (1) and (2) yield n ~ G /(α N 0 ) and βp 2 ~ G (1+ βα −1 p / N 0 ); these expressions are obtained assuming that p, n ≪ N 0 . As we show below, in our structures β ≪ α , therefore, p ~( G / β ) 1/2 , and consequently, n can be expressed as n ~ p ( p / N 0 )( β / α ). The latter relationship suggests that n ≪ p , and therefore, n m ~ p . In this case, photoconduction is dominated by holes and the photoconductivity can be expressed as σ ph,h = eμ h n NC p = eμ h n NC ( G / β ) 1/2 , where μ h is hole mobility and n NC is the density of NCs in the film. As MGB gets filled, the contribution from holes to photoconduction decreases whereas the contribution from electrons increases until the latter reaches the value of σ ph,e = eμ e n NC n = eμ e n NC ( G / α ) 1/2 ( μ e is electron mobility) when the MGB is completely full ( n 0 = N 0 ). The above two limits describe the situations of, respectively, large negative and flat-band gate biases, when the Fermi level is either below or above the MGB ( Fig. 3a ). Because of symmetry between the conduction and valence bands in PbS [28] , [29] , μ e and μ h in our films are likely similar ( μ h ~ μ e = μ ). Therefore, if the electron- and hole-capture probabilities were the same, the filling of the MGB would not lead to changes in total photoconductivity, σ ph = σ ph,e + σ ph,h , as the decrease in σ ph,h would be compensated by the increase in σ ph,e . However, our experimental data ( Figs 1c and 3b ) indicate a decrease in the photoconductivity by a factor ( ξ ) of ca 20 to 50 as V g changes from large negative values to the flat-band voltage. This implies that the electrons provide a smaller contribution to photoconduction than holes and, further, suggests that α is much greater than β . Specifically, in the limits of empty and full MGB, the total photoconductivity can be expressed as σ ph (empty)~ σ ph,h = eμn NC ( G / β ) 1/2 and σ ph (full)= e μ n NC ( G /α) 1/2 + σ ph,h (full), respectively, which yields the ratio ξ = eμn NC ( G / β ) 1/2 /[ e μ n NC ( G /α) 1/2 +σ ph,h (full)]. From this expression, we obtain ( α / β ) 1/2 = ξ [1+ σ ph,h (full) ( eμn NC ) −1 ( α / G ) −1/2 ], which suggests that ( α / β ) 1/2 > ξ . On the basis of the measured ratio of the photocurrents ( Fig. 3b ), we can conclude that α is at least 400 times greater than β . This result indicates that band-edge electrons in our films are much shorter lived than holes ( α ≫ β ) and therefore provide a smaller contribution to the photocurrent. This is probably because of close proximity of the MGB to the conduction band (~0.4 eV versus ~0.9 eV separation from the valence band), which makes trapping through multiphonon emission easier for electrons than for holes [31] . To quantify the relative contributions of band-edge electrons and holes to photoconduction, we solve equations (1) and (2) for the situation when the density of MGB equilibrium charges is much greater than the density of photogenerated carriers ( n 0 ≫ n m and N 0 – n 0 ≫ n m ), and hence, the dynamics of both electrons and holes are controlled by the equilibrium occupancy of the MGB. In this case, σ ph is where u =β/α ≪ 1 and x = n 0 / N 0 . Equation (3) indicates a linear dependence of σ ph on G and it approximates the behaviour of σ ph between the limits of almost complete filling and almost complete depletion of the MGB. The first and the second terms in the right-hand side of equation (3) correspond, respectively, to electron and hole contributions. In Figure 3c , we compare them for β/α=0.002 (black dashed and red dashed-and-dotted lines for holes and electrons, respectively). Interestingly, up to near-unity values of x , the photoconductivity is dominated by valence-band holes and even for x =0.95, the hole contribution to σ ph is more than 20 times greater than that of electrons. This is a direct result of a high capture probability for electrons that quickly relax from the band-edge states into the low-mobility MGB. The short electron lifetime also explains why optical transitions, where MGB electrons are promoted to the conduction band (M' 1S and M' X transitions in Fig. 3a ; red dashed arrows), are not prominent in the photocurrent. The dominant role of hole photoconduction in our devices helps also to rationalize the overall V g -dependent trends observed in the photocurrent spectra ( Fig. 2c ), namely the increase in I sd when V g changes from positive to progressively more negative values. This behaviour reflects the change in the lifetime of photogenerated holes, which becomes progressively longer as MGB gets more depleted of electrons under increasing negative gate bias. Assuming hole-dominated photoconductance, from equations (1) and (2), we can obtain the following expression for σ ph , which in addition to the regime described by equation (3) also allows us to treat the transition to a completely depleted MGB, that is, the range of x from 1 – ɛ to 0 ( ɛ is a small quantity defined by the condition N 0 – n 0 ≫ n m or ɛ ≫ n m / N 0 ): We further use this expression (the corresponding dependence is shown by the blue solid line in Fig. 3c ) to model the measured V g -dependence of photocurrent for different excitation intensities (lines in Fig. 3b ). In our modelling, we relate n 0 to N 0 and V g by where k B is the Boltzmann constant, T is the temperature, and E F = γ ( V g − V 0 ) is the Fermi energy ( γ is the dimensionless constant and V 0 is the flat-band voltage). Equation (5) correctly predicts that under the flat-band condition ( V g = V 0 ), n 0 = N 0 , which corresponds to a fully occupied MGB, and n 0 exponentially decreases for progressively more negative gate voltages. Using equations (4) and (5), we can accurately describe both the gate-voltage and the illumination-intensity dependence of the measured photocurrent ( Fig. 3b ; compare calculations shown by lines with measurements shown by symbols). This confirms the validity of our model and provides an extra piece of evidence that photoconduction in our structures is dominated by valence-band holes. An interesting prediction of equation (4) is that in addition to the magnitude of photoconductivity, the type of light-intensity-dependence of photoconduction can also be controlled by n 0 , and, hence, gate voltage. For example, in the regime of a depleted MGB, when n 0 ≪ 2( G / β ) 1/2 , which realized in our devices for large negative V g , the band-edge electrons quickly relax into the mid-gap states and hole dynamics are dominated by bimolecular recombination with these non-equilibrium MGB electrons. This results in a square-root dependence of σ ph on G : σ ph,h = eμ h n NC ( G / β ) 1/2 . However, as MGB becomes occupied with even a moderate number of electrons ( n 0 ≫ 2( G / β ) 1/2 ), the hole dynamics are dominated by recombination with 'pre-existing' MGB electrons, which leads to a linear dependence of σ ph on G : σ ph,h = eμ h n NC G /( βn 0 ). Our data indeed indicate an approximately square-root scaling of the photocurrent with G for large negative V g ( Fig. 3d ; open red circles). We also observe that the σ ph versus G dependence becomes progressively steeper as V g gets less negative, and the number of MGB electrons increases (compare data shown by solid black squares and open green triangles in Figure 3d ; see also Supplementary Fig. S2 for a different device, which shows a similar change in the scaling of photocurrent with light intensity). This behaviour is consistent with the predicted transition to the linear scaling described by equation (4). The demonstrated control of recombination dynamics by gate voltage is useful in photodetection, where it can be employed for controlling both device sensitivity and its dynamic range. A significant increase in device sensitivity can be obtained by combining contributions from photoconductive and photovoltaic effects. 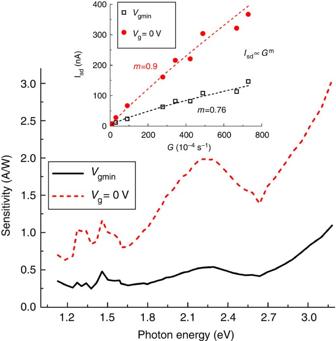Figure 4: Effect of gate bias on OFET sensitivity. Sensitivity (defined as photocurrent per unity incident light intensity) as a function of photon energy at the flat-band voltage (solid black curve; purely photoconductive response) andVg=0 (dashed red curve); 3.1 eV photon energy. The higher sensitivity in the latter case is a result of a combined contribution from the photoconductive and the photovoltaic effects. The contribution from the photovoltaic effect also increases the steepness of the dependence of the photocurrent on photogeneration rate (compare data shown by red solid circles and black open squares in the inset). This is illustrated in Figure 4 (inset) where we compare a purely photoconductive response measured at V g = V gmin (the photocurrent minimum) with one obtained for V g =0; the latter signal exhibits a much faster growth with G due to a photovoltaic contribution. The enhancement in sensitivity arising from the photovoltaic effect is also pronounced in the spectral dependence of a photoresponse (main panel of Fig. 4 ; compare traces shown by solid and dashed lines). Figure 4: Effect of gate bias on OFET sensitivity. Sensitivity (defined as photocurrent per unity incident light intensity) as a function of photon energy at the flat-band voltage (solid black curve; purely photoconductive response) and V g =0 (dashed red curve); 3.1 eV photon energy. The higher sensitivity in the latter case is a result of a combined contribution from the photoconductive and the photovoltaic effects. The contribution from the photovoltaic effect also increases the steepness of the dependence of the photocurrent on photogeneration rate (compare data shown by red solid circles and black open squares in the inset). Full size image The observed difference in hole and electron relaxation times results in a peculiar, mixed character of photoconduction, when holes are transported through quantized states whereas electrons through the MGB. One implication of this transport mechanism is that the photovoltage, which can be derived from such a structure, is determined by the energy difference between the valence-band edge and the MGB. As a result, while displaying correlation with the band-gap energy it should be always lower than the ideal V oc calculated for a given E g . This trend has indeed been observed in NC solar cells [13] , [14] , [15] , [17] , [27] , [32] , [33] ( Supplementary Fig. S3 ). To summarize, we have investigated OFETs fabricated from PbS NCs. Spectrally resolved studies of V g -dependent photocurrent reveal the existence of mid-gap states in NCs films that form a weakly conducting MGB. This band serves as a charge conduit in dark, however, the mechanism of charge transport changes under illumination when it becomes dominated by a more conductive network of quantized band-edge states. In this case, the MGB still has an important role as its occupancy controls photoconduction by controlling recombination dynamics of band-edge charges. 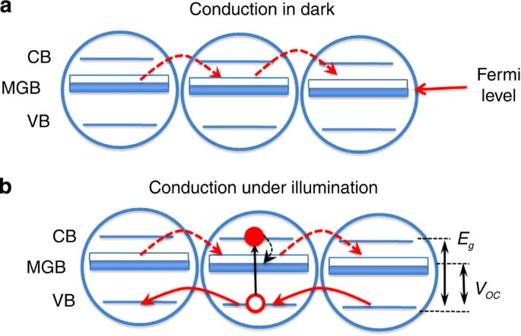Figure 5: Conduction mechanisms in NC films in dark and under illumination. (a) 'Dark' charge transport occurs through a manifold of weakly conductive MGB states. In our films, the MGB is completely full, and hence, insulating under the flat-band condition. Application of a negative gate bias leads to injection of holes into the MGB, which lowers the Fermi level and opens a conducting pathway through the MGB states. (b) The mechanism for charge transport changes under illumination. In this case, the photogenerated electrons get rapidly trapped from the conduction-band (CB) levels into the mid-gap states and are transported through the MGB. On the other hand, photogenerated holes, that are much longer lived, are transported via more-overlapping, highly conductive valence-band (VB) states. Hole transport via the VB levels dominates photoconduction. Because of the 'mixed' character of photoconduction, which involves both the VB and MGB states, the photovoltage is determined not by the intrinsic band-gap energy,Eg, but the VB–MGB separation. The mechanisms for 'dark' and 'light' transport are schematically illustrated in Figure 5 . The results of our studies together with the developed model should help one to predictably engineer both charge transport properties of NC films in dark as well as under illumination. Interesting opportunities could also be opened by engineered placement of MGB states within the NC energy gap. This could allow, for example, switching between electron- and hole-dominated photoconductivity and, perhaps, help in practical realization of advanced photovoltaic concepts such as intermediate-band solar cells [34] . Figure 5: Conduction mechanisms in NC films in dark and under illumination. ( a ) 'Dark' charge transport occurs through a manifold of weakly conductive MGB states. In our films, the MGB is completely full, and hence, insulating under the flat-band condition. Application of a negative gate bias leads to injection of holes into the MGB, which lowers the Fermi level and opens a conducting pathway through the MGB states. ( b ) The mechanism for charge transport changes under illumination. In this case, the photogenerated electrons get rapidly trapped from the conduction-band (CB) levels into the mid-gap states and are transported through the MGB. On the other hand, photogenerated holes, that are much longer lived, are transported via more-overlapping, highly conductive valence-band (VB) states. Hole transport via the VB levels dominates photoconduction. Because of the 'mixed' character of photoconduction, which involves both the VB and MGB states, the photovoltage is determined not by the intrinsic band-gap energy, E g , but the VB–MGB separation. Full size image OFET fabrication PbS NCs with a mean diameter of ca 3.3 nm, were synthesized according to ref. 35 (see transmission electron micrograph in the inset of Fig. 1b ). The NC dispersion was cleaned by repeatedly precipitating and re-dispersing in toluene to remove excess reactants. PbS NCs were then ligand exchanged with oleylamine [33] , and after removal of excess oleylamine, were re-dispersed in octane. The purified NC colloidal suspension in octane was spin-coated onto a doped silicon/silicon-oxide substrate (the oxide layer thickness was ca 100 nm), which served as a gate electrode. This was followed by film treatment with 0.1 M of 1,2-ethanedithiol solution in acetonitrile [14] , and a new spin coating step with the PbS NC suspension and the treatment with 1,2-ethanedithiol. The final thickness of the NC film was ~40 nm, as evaluated from atomic force microscopy measurements. Interdigitated source and drain gold electrodes (50 μm separation) were deposited directly on top of the NC film using a shadow mask. OFET measurements Three-terminal device measurements were conducted using a semiconductor device analyser (B1500A, Agilent Technologies). A constant bias of −25 V was applied between the source and the drain electrodes, while the gate-source bias was varied from 10 to −25 V. In the measurements of the I sd versus V g dependences, we ramped the gate voltage in 1 V increments using three different integration times: t int =640 μs, 16.6 ms, and 267 ms. The measured photocurrent did not vary by more than 5–10% between different values of t int . We also did not detect any difference in traces recorded by ramping the gate either up or down. The light from xenon or tungsten lamps, filtered through a monochromator (~10 nm bandwidth) was used to illuminate the OFET from the top, whereas the photocurrent was monitored as a function of either monochromatic light intensity or incident radiation wavelength. The maximum light intensity incident onto the device was 50 μW cm −2 . Density of charges injected by applying gate voltage We derive the density of charges injected into the channel of the NC–OFET from 'dark' capacitance measurements. The total charge injected for a given gate voltage was calculated from , which yields Q =1.82 μC cm −2 for V g =−25 V. Assuming that, in our devices, NCs form a random close-packed solid, we estimate that the NC surface density per monolayer is ~10 13 cm −2 , which indicates that the average number of charges injected per NC for V g =−25 is ~0.1, assuming that the NC film is ~10-monolayers thick. Density of photogenerated charges Using absorption cross section ( σ abs ) of 10 −15 cm −2 (ref. 36 ) and fluxes ( W ) from 5 to 50 μW cm −2 , we calculate the photogeneration rate, G =( W /ħω) σ abs , from 10 −4 to 10 −6 ms −1 ( ħ ω is photon energy). The lifetime of carriers in our devices ( τ ) is 0.01–1 ms. On the basis of these values, an upper limit of the density of photogenerated charges, n = p = Gτ , is 10 −4 per NC. How to cite this article: Nagpal, P. & Klimov, V.I. Role of mid-gap states in charge transport and photoconductivity in semiconductor nanocrystal films. Nat. Commun. 2:486 doi: 10.1038/ncomms1492 (2011).